One mechanism contributing to co-variability of the Atlantic inflow branches to the Arctic The two-branched inflow of warm and saline Atlantic Water to the Arctic is the major contributor of oceanic heat to the Arctic climate system. However, while the Atlantic Water entering the Arctic through the Fram Strait retains a large part of its heat as it flows along the Arctic continental slope, the branch flowing through the shallow Barents Sea releases a substantial amount of heat to the atmosphere. Hence, the pathway of the Atlantic Water into the Arctic to a large degree determines the short term fate of its heat. Here we show events in which the relative strengths of the two branches are affected by wind-induced Ekman-transport off the northern Barents Sea shelf. The resulting decrease in sea surface height induces a cyclonic circulation anomaly along the slope encircling the northern Barents Sea shelf area, which enhances the flow through the Barents Sea while weakening the branch flowing along the Arctic continental slope. During the last few decades, the Arctic has experienced large climatic changes, for example, reflected in its shrinking ice cover [1] and in increased atmospheric meridional heat transport [2] . In the same period, the Atlantic Water layer in the Arctic has become warmer [3] , [4] . However, it is unclear whether this excessive oceanic heat becomes available for melting sea ice, although some studies report a relation [5] . The two-branched inflow of Atlantic Water to the Arctic has been known for more than a century [6] , [7] . The cooling of the Atlantic Water en route depends strongly on the two pathways towards the Arctic [8] . One branch flows through the Barents Sea and experiences substantial cooling through interaction with the atmosphere. The other branch flows through the Fram Strait, where the warm Atlantic core persists beneath an isolating layer of colder and fresher water masses as it enters the Arctic Ocean [9] ( Fig. 1 ) and flows eastward as a subsurface current along the Arctic continental slope. Thus, the relative strengths of these two Atlantic pathways are potentially key factors in the spatial variability of the Arctic heat budget [10] . Despite their importance and decade-long efforts to monitor these branches in the Barents Sea Opening (BSO) [11] and the Fram Strait [12] , mechanisms that describe how these branches co-vary are lacking. 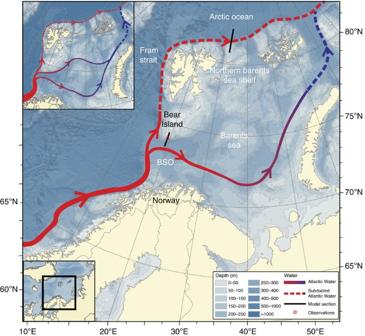Figure 1: Two pathways of Atlantic Water towards the Arctic Ocean. Bathymetric map of the Barents Sea and the general circulation pattern of the Atlantic Water. The inlet shows the main features of the Atlantic Water during circulation anomalies encircling the northern Barents Sea shelf (NBSS), including flow-reversal on the northern slope of the Barents Sea Opening (BSO). Figure 1: Two pathways of Atlantic Water towards the Arctic Ocean. Bathymetric map of the Barents Sea and the general circulation pattern of the Atlantic Water. The inlet shows the main features of the Atlantic Water during circulation anomalies encircling the northern Barents Sea shelf (NBSS), including flow-reversal on the northern slope of the Barents Sea Opening (BSO). Full size image In this study, we provide a mechanistic model of how wind-induced Ekman-transport regulates the co-variation of the two branches of Atlantic Water inflow to the Arctic. The causality is identified and evaluated by a numerical ocean model simulation, using atmospheric reanalysis data and direct current observations on the northern slope of the BSO ( Fig. 1 ). Co-variation in oceanic and atmospheric signals For the southern BSO slope, the estimated volume flux based on current metre moorings is 2.0 Sv [11] compared with the similar model estimate of 2.1 Sv for the period 1998–2008. The new observations, collected on the northern BSO slope not included in the regular monitoring of the BSO and previously only measured during shorter campaigns, together with the ocean model indicate a direct branch of Atlantic Water flowing through the northern Barents Sea and into the Arctic Ocean. According to the ocean model, this coincides with a reduced Atlantic Water flow along the rim of the Arctic Ocean ( Fig. 1 , upper left panel; Fig. 2 ). To substantiate this model result, we found a significant correlation ( R =0.66; P <0.01) between the modelled and the observed depth-averaged currents on the northern slope of the BSO when applying a low-pass filter with a 7-day cutoff period ( Fig. 3a ). The dominant flow direction on the northern slope is towards the west, but it is interrupted by transient flow-reversals. The velocities during such flow reversals, based on the filtered data, reach nearly 0.10 ms −1 , and the observations and the model indicate similar values for both the maximum velocities and the duration of the events. The significant correlation between the modelled and the observed currents justifies using the model simulation to investigate the long-term variability and to identify the forcing of the flow reversals. 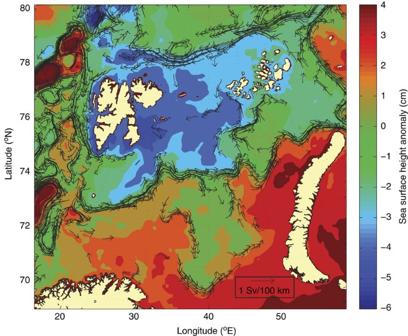Figure 2: Circulation anomaly on the northern Barents Sea shelf (NBSS). Modelled change in de-seasoned monthly mean sea surface height (in colour) and volume transports (arrows) during NBSS circulation anomalies compared with the average over all months. Circulation anomalies are defined to be the months when the de-seasoned ‘h’ estimated by the idealized model (equation (1)) is >1.5 s.d. below the average of all months (12 out of 228 months). The arrows show the corresponding depth-integrated current anomalies (in Sv/100 km width; 1 Sv=106m3s−1), when integrated over the upper 500 m of the water column. Only values above 0.5 Sv/100 km are shown. Figure 2: Circulation anomaly on the northern Barents Sea shelf (NBSS). Modelled change in de-seasoned monthly mean sea surface height (in colour) and volume transports (arrows) during NBSS circulation anomalies compared with the average over all months. Circulation anomalies are defined to be the months when the de-seasoned ‘ h ’ estimated by the idealized model (equation (1)) is >1.5 s.d. below the average of all months (12 out of 228 months). The arrows show the corresponding depth-integrated current anomalies (in Sv/100 km width; 1 Sv=10 6 m 3 s −1 ), when integrated over the upper 500 m of the water column. Only values above 0.5 Sv/100 km are shown. 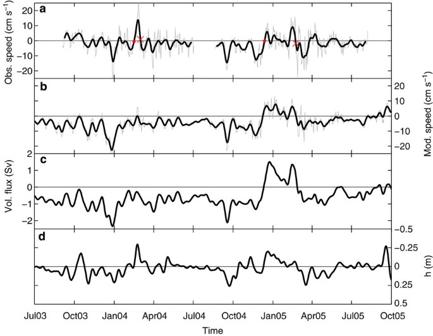Figure 3: Velocity and volume transport along the northern Barents Sea Opening (BSO) slope. (a) Depth-averaged daily (thin lines) and 7-day filtered (thick lines) eastward velocity components from the observations (red bullets and crosses mark start and end, respectively, of periods of major flow-reversal events) and (b) the model in cm s−1; (c) 7-day filtered modelled volume transport along the northern slope of the BSO between 73° 30′N and 74°N in Sverdrup (1 Sv=106m3s−1); (d) 7-day filtered values ofhin metres (note the reversedy-axis). Full size image Figure 3: Velocity and volume transport along the northern Barents Sea Opening (BSO) slope. ( a ) Depth-averaged daily (thin lines) and 7-day filtered (thick lines) eastward velocity components from the observations (red bullets and crosses mark start and end, respectively, of periods of major flow-reversal events) and ( b ) the model in cm s −1 ; ( c ) 7-day filtered modelled volume transport along the northern slope of the BSO between 73° 30′N and 74°N in Sverdrup (1 Sv=10 6 m 3 s −1 ); ( d ) 7-day filtered values of h in metres (note the reversed y -axis). Full size image We therefore use the model results to construct a 19-year time series of the along-slope volume transport on the northern slope of the BSO. This is an integrated measure and chosen in order to reduce the effect of possible displacements of the current up or down the slope. Seeking possible forcing mechanisms, we note that in contrast to the observed baroclinic structure of the mean current, the major observed flow reversals have comparable strength through the entire water column ( Supplementary Fig. S1 ), which suggests a barotropic forcing mechanism. This leads us to investigate relations between the volume transport and the sea surface height in the model simulation. By performing a spatial correlation analysis, we found that the 7-day moving average modelled volume transport for the 19-year period (positive eastward) is anti-correlated with the modelled sea surface height over the entire northern Barents Sea shelf (NBSS) ( R <−0.5; P <0.01; Supplementary Fig. S2 ). This suggests that the flow reversals are local manifestations of a regional pattern. The emergence of such a pattern requires cross-slope volume transport off the shelf, which can be achieved through wind-induced Ekman-transport. With similarities to [13] , we propose that changes in sea surface height over the NBSS to first order is a balance between the integrated Ekman-transport across the rim of the NBSS and a friction term representing for example, bottom Ekman-transport: where h is the areal mean sea surface height over the NBSS, τ is the surface wind stress from the ERA-Interim data set [14] integrated around an idealized box of area A (300,000 km 2 ) along the line s representing the NBSS ( Supplementary Fig. S2 ), ρ s is the density of sea water, f is the Coriolis parameter, and T is a damping time scale set to 1 week. This choice of T is somewhat arbitrary but chosen to obtain a realistic range of sea level variability. Clearly, h , representing the estimated change in sea surface height to changes in wind stress, displays features of variability similar to the modelled volume transport ( Fig. 3c ; R =−0.63; P <0.001, for the 7-day filtered data over the observation period), and to both the observed and modelled eastward velocity components at the northern BSO ( Fig. 3a ). The estimated h is significantly related to the modelled volume transport along the northern slope of the BSO for periods longer than 2–3 days with negligible phase lag ( Supplementary Fig. S3 ). Also, there is a consistent offset in the phase lag such that the Ekman-transport off the NBSS leads the flow. New understanding of how the Barents Sea affects the heat flux to the Arctic A simple interpretation of the above relations is that the wind-induced off-shelf Ekman-transport sets up cross-shelf sea level gradients confined to the continental slope region that generate along-slope current anomalies through geostrophic adjustment. Both observations and the ocean model indicate that the pronounced off-shelf Ekman-transport and flow reversals occur mainly during the winter season. We attribute this tendency to the more vigorous low-pressure activity during winter, with an associated cyclonic wind field over the NBSS. In addition to showing that the northern BSO flow reversals are part of a circulation anomaly encircling the NBSS, we also used the ocean model to quantify the associated changes in volume transports for the two Atlantic inflow branches. We found anomalies of comparable sizes but opposite signs; that is, increase through the BSO (0.8 Sv) and decrease along the Arctic continental slope (−0.9 Sv) and through the entire Fram Strait (−0.6 Sv) during the NBSS circulation anomalies ( Fig. 4 ). Furthermore, the model shows that outflow temperatures in the north-eastern Barents Sea do not change during NBSS circulation anomalies, because of melting of sea ice and increased ocean-to-air heat loss [15] . Therefore, the change in heat flux is basically controlled by the changes in volume flux. Hence, the anomaly circulation corresponds to a reduced oceanic heat transport to the Arctic of about 10 TW based on a model temperature difference of 3.2 °C between the core of the Arctic Continental slope branch (2.4 °C) and the north-eastern Barents Sea outflow (−0.8 °C). Corresponding observed mean temperatures are 2.5 °C (ref. 16 ) and −0.5 °C (ref. 17 ). In general, the Atlantic Water inflow through the BSO is located on the southern slope [18] , while the Arctic Water outflow is limited to the northern slope ( Fig. 4a ). During periods of northern BSO flow-reversal, inflowing Atlantic Water suppresses the Arctic Water up-slope and continues along the southern slope of the NBSS ( Fig. 2 ). According to the model this constitutes the southern limb of the NBSS circulation anomaly. 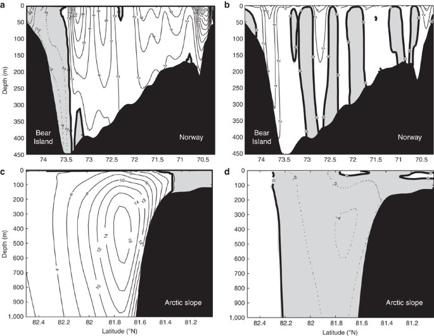Figure 4: Vertical sections of velocities and velocity anomalies. (a) Modelled average velocity through the Barents Sea Opening (BSO); (b) velocity anomalies through the BSO during northern Barents Sea Shelf (NBSS) circulation anomaly events; (c) modelled average velocity through the Arctic slope section; (d) velocity anomalies through the Arctic slope section during NBSS circulation anomaly events. Averages are based on all months in the period 1990–2008, with positive values toward the east. Anomalies are averages for all months when ‘h’ is >1.5 s.d. below its mean value. The seasonal signal is compensated for when calculating the anomalies by subtracting the long-term average for each month separately. Figure 4: Vertical sections of velocities and velocity anomalies. ( a ) Modelled average velocity through the Barents Sea Opening (BSO); ( b ) velocity anomalies through the BSO during northern Barents Sea Shelf (NBSS) circulation anomaly events; ( c ) modelled average velocity through the Arctic slope section; ( d ) velocity anomalies through the Arctic slope section during NBSS circulation anomaly events. Averages are based on all months in the period 1990–2008, with positive values toward the east. Anomalies are averages for all months when ‘ h ’ is >1.5 s.d. below its mean value. The seasonal signal is compensated for when calculating the anomalies by subtracting the long-term average for each month separately. Full size image Our investigation of the proposed forcing mechanism is simplified. First, complex atmosphere-ocean interactions are represented by wind-induced Ekman-transport and subsequent response in sea surface height on the NBSS. Second, the NBSS circulation anomaly described here is superimposed onto the upstream variability of Atlantic Water flow towards the Arctic (for example, refs 12 , 19 ). Despite these simplifications, we still find that the estimated wind-driven off-shelf Ekman-transport and subsequent response in sea surface height can explain a statistically significant part of the modelled NBSS circulation anomaly and its manifestation on the northern slope of the BSO. This suggests that the proposed mechanism is a robust feature of the Atlantic water pathways into the Arctic. The North Atlantic Oscillation (NAO) [20] impacts the Arctic through interannual and decadal changes in the storm tracks in the Nordic Seas [21] . Although acting on a larger scale, the result is a northerly shift in storm tracks during a positive phase of the NAO [22] and likely a change in the frequency of NBSS circulation anomalies. Indeed, such events were more frequent during the 1990s coinciding with a high NAO state compared with the 2000s when the NAO was fluctuating around its average. In a warming climate, the NAO is expected to become more positive [23] , and the northern hemisphere storm tracks are expected to shift northwards [24] potentially affecting the relative strength of the Atlantic Water pathways and thereby also the oceanic heat transport to the Arctic through the suggested mechanism described here. Overall, the total oceanic heat advection to the Arctic will change depending on both the total flow of Atlantic Water towards Arctic and the distribution between the Barents Sea and Fram Strait branches. Hence, the proposed mechanism, where wind-induced Ekman-transport off the NBSS regulates the relative strength of the two Atlantic Water pathways to the Arctic, represents one key element of importance when assessing how climate change will affect the Arctic. Current measurements A 75-kHz RDI WorkHorse LongRanger Acoustic Doppler Current Profiler was deployed to the south of Bear Island at 73°N 51′, 19°E 15′ ( Fig. 1 ) for two consecutive years from September 2003 to August 2005. The instrument sampled velocities every 20 min at an 8-m-bin vertical resolution covering the full water column. The water depth in the deployment area is 220 m, and the bathymetry is oriented east–west. The measurements were smoothed with a 25-h moving average to exclude tides and then resampled every 24 h to represent daily averages. There was an ∼ 10° difference in mean velocity direction between the two deployment periods. The cause of this difference, which may have been due to compass errors or small-scale topographic effects, has not been resolved. However, this error is small relative to the flow reversals that are the main focus here, and therefore, it does not influence the main results. Atmospheric data Monthly averages of the surface wind stress components in the Barents Sea region were obtained from the ERA-Interim reanalysis [14] for the period from 1990 to 2008 at a spatial resolution of 1.5 by 1.5 degrees. Numerical model The Regional Ocean Modelling System (ROMS) was run on a 4 by 4 km horizontal resolution grid covering the Nordic, Barents and Kara seas [25] . ROMS is a three-dimensional baroclinic ocean general circulation model that uses normalized, topography-following sigma coordinates in the vertical direction [26] . The simulation was performed for the period from 1989 to 2008, but in the analysis, we discarded 1989 as a model spin-up year. The model was forced at the lateral open boundaries by monthly averages from a global simulation with ROMS using a similar model setup but at a coarser horizontal grid resolution. Atmospheric forcing was taken from 6-h ERA-Interim reanalysis data [14] that included wind stress, sea level pressure, short- and long-wave radiation and precipitation. An ice module was coupled with the model [27] , and velocities and amplitudes from eight tidal constituents derived from the Arctic Ocean Tidal Inverse Model [28] were imposed at the lateral open boundaries. From the modelled data archive, we computed the daily mean eastward velocity component in the model grid point closest to the location of the observations. In addition, daily averaged volume transports were computed through a section that covers the northern slope of the BSO and passes through the observation site, as well as monthly averaged volume transport through the entire BSO. Mean modelled volume flux in the BSO for the period 1998–2008 covered by moorings is 2.1 Sv compared with observations indicating 2.0 Sv [11] . Estimate of volume transport anomalies The modelled volume transports in the two inflow branches were calculated through sections in the BSO (70° 10′N, 20°E–74°20′N, 19° 30′E), the Fram Strait (79° 24′N, 10°W–79° 24′N, 10° 30′E) and on the Arctic continental slope (81°N–82° 30′N, 31°E), while volume transport on the northern BSO slope was calculated through a sub-section from 73° 30′N–74°N, 19°E ( Fig. 1 ). In the BSO and Fram Strait, we have calculated net transport (eastward/northward minus westward/southward) for all water masses flowing through the sections. On the Arctic continental slope, the challenge is to include only relevant water masses. We have chosen to define the Arctic Circumpolar Boundary Current carrying Atlantic Water as the region where the velocity is larger than the e-folding of the maximum velocity in the core of the flow: where e is the natural logarithm. However, this flow includes both Atlantic Water and a mixture of diluted Atlantic Water and the basin circulation in the Polar Basin. Hence, the mean volume transport (8.3 Sv) is larger than the upstream core of Atlantic flow. The volume transport anomalies are de-seasoned monthly mean changes during NBSS circulation anomalies (h >1.5 s.d. below the average of all months) compared with the average of all months. How to cite this article: Lien, V. S. et al. One mechanism contributing to co-variability of the Atlantic inflow branches to the Arctic. Nat. Commun. 4:1488 doi: 10.1038/ncomms2505 (2013).